Haemodynamically dependent valvulogenesis of zebrafish heart is mediated by flow-dependent expression ofmiR-21 Heartbeat is required for normal development of the heart, and perturbation of intracardiac flow leads to morphological defects resembling congenital heart diseases. These observations implicate intracardiac haemodynamics in cardiogenesis, but the signalling cascades connecting physical forces, gene expression and morphogenesis are largely unknown. Here we use a zebrafish model to show that the microRNA, miR-21 , is crucial for regulation of heart valve formation. Expression of miR-21 is rapidly switched on and off by blood flow. Vasoconstriction and increasing shear stress induce ectopic expression of miR-21 in the head vasculature and heart. Flow-dependent expression of mir-21 governs valvulogenesis by regulating the expression of the same targets as mouse/human miR-21 ( sprouty , pdcd4 , ptenb ) and induces cell proliferation in the valve-forming endocardium at constrictions in the heart tube where shear stress is highest. We conclude that miR-21 is a central component of a flow-controlled mechanotransduction system in a physicogenetic regulatory loop. Formation of the three-dimensional structure of the heart begins with fusion of bilateral mesodermal planes that subsequently differentiate into beating cardiomyocytes [1] , [2] . Initially, the cardiomyocytes contract randomly but they soon become synchronized as the heart tube develops. Subsequently, the contractions are coordinated into rhythmic waves along the heart tube generating unidirectional blood flow. In the early valveless stages, one-way flow is generated by a hydroelastic suction pump [3] . Later, an S-shaped bend forms in the tube and the cardiomyocytes proliferate causing bulges, which develop into two distinct chambers, the atrium and ventricle, with constrictions in the outflow tract (OFT) and atrioventricular (AV) canal. Valves develop at these strictures to ensure unidirectional circulation. Throughout these morphogenetic events, blood flow is maintained. As the valves form at constrictions, the valve-forming endocardial cells are subject to higher sheer forces. Many studies have suggested that haemodynamic stresses provide essential morphogenetic cues for normal cardiogenesis. Perturbation of blood flow by beads in zebrafish heart causes morphological defects like those observed in congenital heart diseases [4] , [5] . Auman et al. [6] reported that the blood flow and contractility regulate the shape of cardiomyocytes and the form of the heart. More recently, reversing blood flow has been shown to regulate valvulogenesis via expression of krüppel-like factor 2a ( klf2a ) (ref. 7 ), highlighting a putative link between gene expression and mechanical stimuli. MicroRNAs (miRNAs) are small non-coding RNAs. Primary transcripts of miRNAs are processed by Drosha and Dicer and the products are incorporated into the RNA-induced silencing complex [8] . Target mRNAs are degraded or repressed at the translational level, bypassing the transcriptional control of mRNA [9] . We speculated that this rapid regulation might be active during cardiogenesis to couple morphogenesis with haemodynamic changes. This idea is further supported by reports that several miRNAs are induced in mouse hearts subjected to pressure overload [10] and in mechanically stretched smooth muscle [11] . Moreover, recent studies have suggested that miRNAs contribute to haemodynamically dependent cardiogenesis [12] and angiogenesis [13] . miR-21 is highly expressed in malignant tissues and has several target genes, including PDCD4 , PTEN and SPRY2 . These genes exhibit a tumour-suppressing effect, classifying it as an oncomiR [14] . Accordingly, deletion of mouse miR-21 suppresses lung tumorigenesis by modulating the Ras/MEK/ERK pathway and apoptosis [15] . miR-21 is also expressed during cardiac remodelling and appears to be functional in cardiovascular diseases [16] . However, stress-induced cardiac remodelling occurs in the absence of miR-21 in the mouse [17] . In this report, we provide evidence that miR-21 functions differently in zebrafish. By sensing blood flow, it regulates heartbeat-dependent valvulogenesis by repression of the same target genes as in the mouse. We conclude that miR-21 is a crucial component of the programme that regulates valve formation in the zebrafish heart, using haemodynamic stimuli as a physical morphogen. Expression patterns of zebrafish miR-21 In zebrafish, valvulogenesis is initiated between 24 and 48 h post-fertilization (hpf) at the AV canal [18] . Within the canal, the pulsatile flow has critical roles for multiple morphogenetic events, including cell shape changes, protrusion of valve leaflets and expression of klf2a (ref. 7 ). Expression of miR-21 started at 36 hpf in a small subset of the endocardial cells at the AV constriction ( Fig. 1a ). At 48 hpf, this expression became stronger with an additional endocardial spot in the OFT ( Fig. 1b ). These two domains became evident at 72 hpf. The expression patch in the AV canal developed a hole at the centre corresponding to the lumen, while the OFT expression exhibited a streak parallel to the blood flow ( Fig. 1c ). miR-21 expression in the AV canal was restricted to the endocardial cells and was not observed in the myocardium ( Fig. 1d ). As cardiogenesis proceeded, similar expression patterns were observed at 120 hpf ( Fig. 1e ), and even in the valves of more than 1-year-old adult fishes ( Fig. 1f ). The expression patterns are summarized in Fig. 1h . 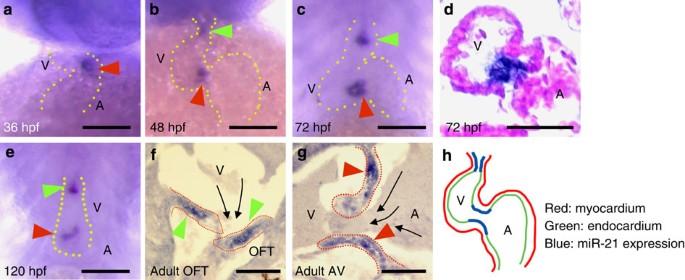Figure 1: Expression patterns ofmiR-21. (a) Soon after initiation of blood flow (36 hpf),miR-21began to be expressed in a subset of the endocardial cells in the AV canal (red arrowhead). A, atrium; V, ventricle. (b) At 48 hpf, endocardial expression in the OFT became evident (green arrowhead). Expression at the AV canal was arranged around the canal lumen (red arrowhead). (c,d) The same expression patterns were maintained at 72 hpf (c) and 120 hpf (e). (d) In sections,miR-21expression was detected only in the endocardial cells, not in the myocardial layer. (f,g) Expression ofmiR-21was detected in the valves of adult fish at the OFT (green arrowheads inf) and the AV canal (red arrowheads ing). Dotted red lines indicate contours of the valves. Black arrows indicate the direction of blood flow. (h) A schematic representation ofmiR-21expression only in specific regions of the endocardium of the OFT and the AV canal (blue lines). Scale bars, 50 μm. Figure 1: Expression patterns of miR-21 . ( a ) Soon after initiation of blood flow (36 hpf), miR-21 began to be expressed in a subset of the endocardial cells in the AV canal (red arrowhead). A, atrium; V, ventricle. ( b ) At 48 hpf, endocardial expression in the OFT became evident (green arrowhead). Expression at the AV canal was arranged around the canal lumen (red arrowhead). ( c , d ) The same expression patterns were maintained at 72 hpf ( c ) and 120 hpf ( e ). ( d ) In sections, miR-21 expression was detected only in the endocardial cells, not in the myocardial layer. ( f , g ) Expression of miR-21 was detected in the valves of adult fish at the OFT (green arrowheads in f ) and the AV canal (red arrowheads in g ). Dotted red lines indicate contours of the valves. Black arrows indicate the direction of blood flow. ( h ) A schematic representation of miR-21 expression only in specific regions of the endocardium of the OFT and the AV canal (blue lines). Scale bars, 50 μm. Full size image Haemodynamically dependent expression of zebrafish miR-21 The presence of miR-21 expression at constricted sections of the endocardium suggested that it might be influenced by the blood flow. To investigate this, heartbeat was stopped by injecting a morpholino antisense oligonucleotide (MO) against troponin T2 ( tnnt2 ) (refs 18 , 19 ). In this morphant, expression of miR-21 was not observed at either 48 or 72 hpf ( Fig. 2b ), whereas beating hearts showed distinct two expression spots ( Fig. 2a ). 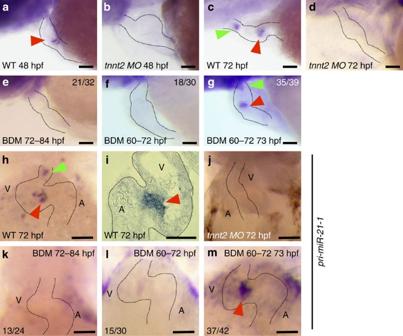Figure 2: Effect of heartbeat on expression ofmiR-21in the developing heart tube. (a,c) Normal expression ofmiR-21at the OFT (green arrowhead) and the AV canal (red arrowheads) at 48 (a) and 72 hpf (c). Dotted lines outline the heart. (b,d). In thetnnt2morphants, expression ofmiR-21was detected neither at 48 (b) nor at 72 hpf (d). (e–g) Twelve hours arrest of heartbeat (from 72 to 84 hpf ine, and from 60 to 72 hpf inf) obliterated the two patches ofmiR-21expression, whereas just 1 h of heartbeat restored the full expression (g). (h–m)pri-miR-21-1transcripts were expressed in the same patterns at 72 hpf (whole mount inh, and section ini). This expression was lost in thetnnt2morphant heart (j). Expression ofpri-miR-21disappeared after 12 h cardiac arrest (from 72 to 84 hpf ink, and from 60 to 72 hpf inl) and 1 h of heartbeat restored it (red arrowhead inm). WT, wild type; MO, morphant; BDM, treated with BDM. Scale bars, 50 μm. Figure 2: Effect of heartbeat on expression of miR-21 in the developing heart tube. ( a , c ) Normal expression of miR-21 at the OFT (green arrowhead) and the AV canal (red arrowheads) at 48 ( a ) and 72 hpf ( c ). Dotted lines outline the heart. ( b , d ). In the tnnt2 morphants, expression of miR-21 was detected neither at 48 ( b ) nor at 72 hpf ( d ). ( e – g ) Twelve hours arrest of heartbeat (from 72 to 84 hpf in e , and from 60 to 72 hpf in f ) obliterated the two patches of miR-21 expression, whereas just 1 h of heartbeat restored the full expression ( g ). ( h – m) pri-miR-21-1 transcripts were expressed in the same patterns at 72 hpf (whole mount in h , and section in i ). This expression was lost in the tnnt2 morphant heart ( j ). Expression of pri-miR-21 disappeared after 12 h cardiac arrest (from 72 to 84 hpf in k , and from 60 to 72 hpf in l ) and 1 h of heartbeat restored it (red arrowhead in m ). WT, wild type; MO, morphant; BDM, treated with BDM. Scale bars, 50 μm. Full size image Silent heart mutants ( sih ), in which tnnt2 is mutated, exhibit morphological defects in their hearts. To exclude the possibility that the loss of the miR-21 expression in the tnnt2 morphants was a secondary effect of those abnormalities, we stopped the heartbeat temporarily and reversibly using 2,3-butanedione monoxime (BDM, a myosin ATPase inhibitor) [20] . When the heartbeat was arrested for 12 h, from 72 to 84 hpf, expression of miR-21 was suppressed at 84 hpf (in 21 of 32 fish, Fig. 2e ). Similarly, when the heartbeat was stopped from 60 to 72 hpf, expression was lost at 72 hpf (in 18 of 30 fish, Fig. 2f ). These data indicate that arrest of the heartbeat for 12 h is sufficient to cancel expression of miR-21 . Conversely, when the heartbeat was reinitiated by washing out the BDM at 72 hpf, miR-21 expression was reestablished at 73 hpf at both valve-forming regions (in 35 of 39 fish, Fig. 2g ). Thus, beating for 1 h can restore the full expression. Biogenesis of mature miRNAs is regulated at multiple steps from transcription of primary miRNAs to the RNA-induced silencing complex-mediated targeting to mRNAs [21] . To check a transcriptional control of miR-21 , we made a probe that specifically recognizes pri-miR-21-1 , one of two primary transcripts of zebrafish miR-21 on two different chromosomal loci. At 72 hpf, this probe localized at the same positions ( Fig. 2h ). In sections, expression of pri-miR-21-1 was observed in the valve-forming endocardial cells ( Fig. 2i ). It was absent in the tnnt2 morphants at 72 hpf ( Fig. 2j ). Similarly, 12 h of arrest cancelled the expression at 84 and 72 hpf (13 of 24 and 15 of 30 fishes, respectively, Fig. 2k ), and 1 h of heartbeat restored it (37 of 42 fishes, Fig. 2m ). These data indicate that transcription of pri-miR-21 is regulated in a heartbeat-dependent manner and that the transcriptional response to heart beating is very fast. It has been shown that the valve formation is dependent on the retrograde flow, rather than blood viscosity, as verified in gata1 and gata2 morphants [7] . The gata1 morphants lack circulating blood cells [22] , hence have lower blood viscosity, whereas the gata2 morphants have reduced retrograde flow at the AV canal [7] , due to abnormal vascular development [23] . Valve formation was selectively impaired in the gata2 morphants with a loss of klf2a expression. In accordance, expression of miR-21 was lost in the gata2 morphants, not in the gata1 (see Supplementary Fig. S1 ), supporting the importance of the reversing flow. In addition, injection of MO against neither klf2a nor tbx2b abrogated the expression of miR-21 . This suggests independence of the miR-21 expression from klf2a or the AV boundary formation in the myocardium [24] (see Supplementary Fig. S1 ). In an opposite approach, we bathed embryos in water containing 2 mM epinephrine at 51.5 hpf for 1.5 h to elevate the heart rate along with vasoconstriction. This stimulation should increase the mechanical stress to the valve-forming endocardial cells and the vascular endothelium in the periphery. After the stimulation, the expression of pri-miR-21-1 in the valve was slightly intensified ( Fig. 3b ), relative to the normal expression ( Fig. 3a ). In the tnnt2 morphants, the expression was repressed, even in the presence of epinephrine ( Fig. 3e ). Next, we injected MO against gata1 , which eliminated blood cells [22] and lowered the viscosity [7] . The expression of pri-miR-21-1 was not affected ( Fig. 3c ) and, in the stimulated heart, this expression was enhanced ( Fig. 3d ). 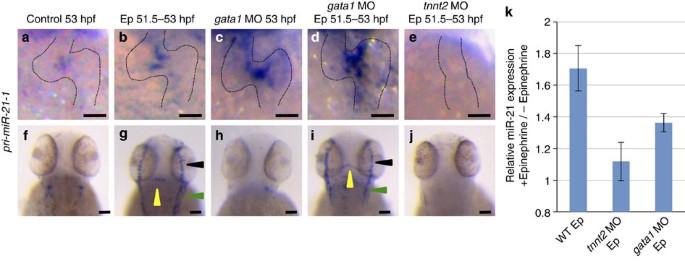Figure 3: Expression patterns ofpri-miR-21-1,the primary transcript ofmiR-21. Expression ofpri-miR-21-1in the heart (a–e) and the head vasculature (f–j) at 53 hpf. The WT (a,b,fandg),gata1morphants (c,d,handi) andtnnt2morphants (e,j) were stimulated by epinephrine (Epi) from 51.5 to 53 hpf (b,d,e,g,iandj). Without Epi stimulation,pri-miR-21-1was expressed only in the valve-forming endocardium (a), not in the head vasculature (f). Elimination of blood cells from the circulation by knocking downgata1did not affect the expression (c,h). After stimulation by Epi, expression ofpri-miR-21-1became slightly stronger at the AV canal (b). (g) Expression in the head became evident in the metencephalic artery/middle cerebral vein (yellow arrowheads), the primary head sinus (green arrowheads) and the primordial mid-brain channel (black arrowheads). This ectopic induction was not affected in thegata1morphants (i), but the absence of heartbeat cancelled it (j). (k) Relative expression of the maturemiR-21was measured by qRT–PCR using RNA isolated from the whole bodies. In the WT, Epi induced ~1.7-fold, whereas the induction in thetnnt2morphant was minimal. In thegata1morphants,miR-21was induced at a relatively lower extent than the WT (~1.4-fold). Scale bars, 50 μm (a–e), 100 μm (f–j). Figure 3: Expression patterns of pri-miR-21-1, the primary transcript of miR-21 . Expression of pri-miR-21-1 in the heart ( a – e ) and the head vasculature ( f – j ) at 53 hpf. The WT ( a , b , f and g ), gata1 morphants ( c , d , h and i ) and tnnt2 morphants ( e , j ) were stimulated by epinephrine (Epi) from 51.5 to 53 hpf ( b,d,e,g,i and j ). Without Epi stimulation, pri-miR-21-1 was expressed only in the valve-forming endocardium ( a ), not in the head vasculature ( f ). Elimination of blood cells from the circulation by knocking down gata1 did not affect the expression ( c , h ). After stimulation by Epi, expression of pri-miR-21-1 became slightly stronger at the AV canal ( b ). ( g ) Expression in the head became evident in the metencephalic artery/middle cerebral vein (yellow arrowheads), the primary head sinus (green arrowheads) and the primordial mid-brain channel (black arrowheads). This ectopic induction was not affected in the gata1 morphants ( i ), but the absence of heartbeat cancelled it ( j ). ( k ) Relative expression of the mature miR-21 was measured by qRT–PCR using RNA isolated from the whole bodies. In the WT, Epi induced ~1.7-fold, whereas the induction in the tnnt2 morphant was minimal. In the gata1 morphants, miR-21 was induced at a relatively lower extent than the WT (~1.4-fold). Scale bars, 50 μm ( a – e ), 100 μm ( f – j ). Full size image Although the endothelial cells in the head do not express pri-miR-21-1 ( Fig. 3f ), they exhibited strong expression after the epinephrine treatment ( Fig. 3g ). This induction was not cancelled by injection of the gata1 MO ( Fig. 3i ). In the tnnt2 morphants, pri-miR-21-1 was not expressed in the head, even after the epinephrine stimulation ( Fig. 3j ). Injection of the gata1 MO alone did not induce pri-miR-21-1 ( Fig. 3h ). To confirm further, we semi-quantitated the expression of miR-21 by quantitative real-time PCR (qRT–PCR) on RNA isolated from the whole bodies ( Fig. 3k ). The epinephrine treatment induced miR-21 ~1.7-fold in the WT and 1.4-fold in the gata1 MO. As expected, this induction was cancelled in the tnnt2 . Haemodynamic parameters were measured in the middle cerebral vein before and after the adrenergic stimulation (see Supplementary Fig. S2 ). The shear stress was estimated to be increased 2.1-fold by epinephrine. Physical regulation of miR-21 expression was confirmed using cultured mammalian cells (see Supplementary Fig. S2 ). Application of 2.0 Pa of shear stress (equivalent to that at the luminal surface of the human aorta [25] ) with a unidirectional laminar flow over human umbilical vein endothelial cells (HUVECs) rapidly induced expression of mature miR-21 . The primary miR-21 transcript was induced more strongly. KLF2 was induced rapidly within 15 min, and the expression increased progressively, hitting the highest peak after 2 h. These results indicate that a set of genes can be induced by the shear stress, but with different temporal profiles. We have found another valve-specific gene, egr1 , which expression is dependent on the heartbeat (see Supplementary Fig. S2 ). Previously, we have reported that myocardial expression of miR-143 in the OFT is dependent on the heartbeat [12] . Nonetheless, induction of miR-143 by mechanical stresses is slower. This suggests that the adaptive responses triggered by the mechanical stimuli are temporally controlled. Laminar flow has been shown to induce other genes in HUVECs (including Klf2, COX-2 , ICAM-1 and c-fos ) [26] , [27] , but the response of miR-21 is the fastest. In addition to the temporal control, cells react differentially to different flows, such as laminar versus turbulent flows and unidirectional versus reciprocating ones [28] . pri-miR-21 was induced more rapidly when reciprocating flow at 0.5 Hz was applied, although induction of mature miR-21 was kept weak (see Supplementary Fig. S2 ). In this condition, Klf2 was also induced faster, but weakly than the unidirectional flow. Induction of pri-miR-21 was sustained longer. 1.0 Hz reciprocating flow exerted the similar effect, but induction of pri-miR-21 was more robust. Interestingly, induction of mature miR-21 was very weak in HUVECs stimulated by the reciprocating flow. This suggests that processing of pri-miR-21 might be repressed by this flow. This also implies that the actions of miR-21 might be repressed even after stimulation by specific shear stress, consistent with the fact that genetic deletion of miR-21 does not affect the correct formation of vasculature and heart [15] . A valveless phenotype of miR-21 morphants To explore the roles of miR-21 , we injected MOs of several designs against miR-21 at the one-cell stage ( Fig. 4 ) (see Methods). For this experiment, we designed two types of MOs, one for multiblocking that disturbs both Dicer and Drosha-mediated processing and another for Guide Dicer that masks guide sequence to block processing miR-21-1 and miR-21-2 by Dicer. These MOs gave similar results. Co-injection of both miR-21-1 and miR-21-2 MOs knocked down miR-21 more efficiently. The expression of miR-21 in the morphants was reduced to one-third of that in the WT (see Supplementary Fig. S3 ). Scrambled MO did not induce obvious abnormalities ( Fig. 4b ). At 48 hpf, blood pooled on the surface of the yolk in the morphants indicating stagnation of flow ( Fig. 4c ). The hearts of the morphants are narrower, showing incomplete looping (Fig. 4g,h). Other parts of body were normal, except for slight hypoplasia of the hindbrain, where miR-21 was weakly expressed. 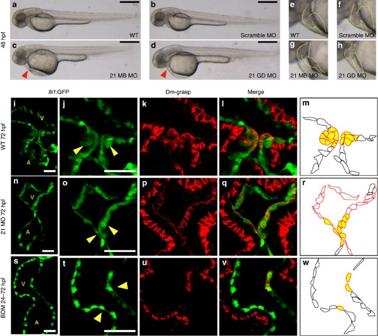Figure 4: A valvelessmiR-21morphant. (a–d) Blood flow of themiR-21morphants stagnated with pooling of blood cells on the yolk at 48 hpf (red arrowhead inc,d) (MB, multiblocking MO; GD, Guide Dicer MO). This stagnation was neither present in the WT (a) nor embryos injected with a scrambled MO (b). Higher magnification views are shown ine–h, with heart contours indicated by dotted lines. (i–m) At 72 hpf, thick layers of the GFP-positive endocardial cells were protruded into the AV canal (i), with cuboidal thickening cells (yellow arrowheads inj). Cell shapes are visualized by Dm-grasp staining (k,l). Dm-grasp- and GFP-positive cells are cuboidal, whereas Dm-grasp-negative and GFP-positive cells are squamous (l). (m) A schematic representation of the endocardial cells, with cells in the valve-forming area shown in yellow, Dm-grasp-positive cells in red lines, negative cells in black lines, respectively. A, atrium, V, ventricle. (n–r) In themiR-21morphants, only a thin layer of endocardial cells was evident with neither thickening nor protrusion into the lumen. (s–w) When heartbeat was stopped from 24 to 72 hpf by BDM, neither thickening nor protrusion of the endocardium was initiated. The number of the Dm-grasp-positive endocardial cells was reduced. Scale bars, 500 μm (a–d), 50 μm (i,j,n,o,s,t). Figure 4: A valveless miR-21 morphant. ( a – d ) Blood flow of the miR-21 morphants stagnated with pooling of blood cells on the yolk at 48 hpf (red arrowhead in c , d ) (MB, multiblocking MO; GD, Guide Dicer MO). This stagnation was neither present in the WT ( a ) nor embryos injected with a scrambled MO ( b ). Higher magnification views are shown in e – h , with heart contours indicated by dotted lines. ( i – m ) At 72 hpf, thick layers of the GFP-positive endocardial cells were protruded into the AV canal ( i ), with cuboidal thickening cells (yellow arrowheads in j ). Cell shapes are visualized by Dm-grasp staining ( k , l) . Dm-grasp- and GFP-positive cells are cuboidal, whereas Dm-grasp-negative and GFP-positive cells are squamous ( l ). ( m ) A schematic representation of the endocardial cells, with cells in the valve-forming area shown in yellow, Dm-grasp-positive cells in red lines, negative cells in black lines, respectively. A, atrium, V, ventricle. ( n – r ) In the miR-21 morphants, only a thin layer of endocardial cells was evident with neither thickening nor protrusion into the lumen. ( s – w ) When heartbeat was stopped from 24 to 72 hpf by BDM, neither thickening nor protrusion of the endocardium was initiated. The number of the Dm-grasp-positive endocardial cells was reduced. Scale bars, 500 μm ( a – d ), 50 μm ( i,j,n,o,s,t ). Full size image In sections, the clustering and thickening of the valve-forming cells, visualized by fli1:GFP [29] and Dm-grasp staining [30] , were absent in the morphants at 72 hpf ( Fig. 4n–r ), whereas those are obvious in the WT ( Fig. 4i–m ). These changes were also lost in the hearts arrested from 24 to 72 hpf by BDM ( Fig. 4s–w ). Although the similar abnormalities in the endocardium were evident at 55 hpf, myocardial cell shape change in the AV canal occurred normally in the morphants. (see Supplementary Fig. S4 ). Further verification was provided by rescue experiments using miR-21 duplex (see Supplementary Fig. S3 ). As there were fewer valve-forming cells in the morphants, we counted their numbers, and found significant reductions in both the miR-21 morphants and the BDM-treated hearts, without affecting the myocardial cells (see Supplementary Fig. S3 ). In addition, expression of proliferating cell nuclear antigen (PCNA) [31] was lost or weak in the valve-forming cells in the miR-21 morphants and embryos treated with BDM (see Supplementary Fig. S5 ). We examined the expression of several markers. Specification of the atrial versus ventricular identity was not affected (see Supplementary Fig. S3 ). In addition, expression of two myocardial markers was not affected by the miR-21 MO, although expression of versican was expanded (see Supplementary Fig. S6 ). Expression of two markers for the valve-forming endocardial cells, hyaluronan synthase 2 ( has2 ) and notch1b , was observed widely in both the atrial and the ventricular compartments (see Supplementary Fig. S6 ). Flow-dependent expression of egr1 was severely reduced [32] , probably due to weak blood flow in the miR-21 morphants (see Supplementary Fig. S6 ). Expression of the secreted phosphoprotein 1 ( spp1 ), the endocardial marker at later stages of the valve development, was reduced, suggesting that maturation of valves was impaired. This decline might be partially due to the weak expression of egr1 , as Spp1 was reported to be a direct target of Egr1 in mouse and GC-rich Egr1-binding motifs are conserved in spp1 (ref. 33 ). As shown later, a loss of function of miR-21 results in reduction of the mitogen-activated protein (MAP) kinase cascade. As the MAK kinase signals were shown to be involved in the expression of Egr1 (ref. 34 ), this pathway could modulate expression of egr1 in zebrafish. Expression of klf2a was not affected. Sprouty 2 as a target of miR-21 As a member of the oncomiRs, miR-21 has been analysed in mammals, and several targets identified [14] , [35] . Sprouty2 ( spry2 ), which encodes a potent inhibitor of the RTK/Ras/ERK pathway, is a direct target [36] , [37] . An exhaustive search of three databases (miRbase, RNAi web and BiBiServ) revealed no new targets but confirmed spry2 in zebrafish. As shown in Fig. 5a , the seed sequence of zebrafish miR-21 shows significant paring at its 5′-end (see Supplementary Fig. S7 ). To verify further, we synthesized two mRNAs. The first mRNA encoded enhanced green fluorescent protein (EGFP) with a 3′-untranslated region (UTR) of spry2 and the other encoded mCherry fluorescent protein with a poly(A) signal alone. When these mRNAs were injected along with the miR-21 MO, both green and red fluorescent signals were detected (left panel, Fig. 5b ). However, when a synthesized duplex of miR-21 was co-injected, EGFP signals was selectively repressed (middle panel, Fig. 5b ), indicating that translation of EGFP was inhibited by the miR-21 duplex. When the seed sequence in the 3′-UTR of spry2 was mutated, EGFP signals were not repressed (right panel, Fig. 5b ). 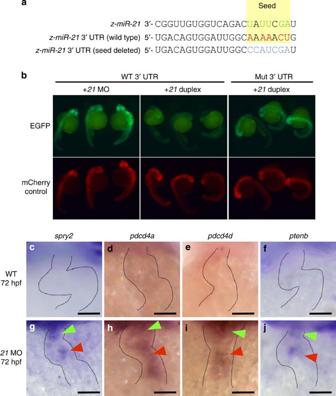Figure 5: Sequence alignment and expression patterns of selected genes. (a) Sequence alignment of zebrafishmiR-21, 3′-UTR ofspry2and its mutated version is shown, with the seed sequences highlighted in yellow and the complementary nucleotides in red and green. (b) TheEGFP-spry2reporter with the WTspry23′-UTR gave strong fluorescent signals when the endogenousmiR-21was blocked by the MO against it (left panel), but failed to show the signals when co-injected with themiR-21duplex (middle panel). TheEGFP-spry2reporter mRNA, in which the seed sequence was mutated, produced strong signals even when co-injected with themiR-21duplex (right panel) at 24 hpf. (c,g) Expression of the endogenousspry2was not observed in the WT at 72 hpf (c), whereas it was induced in both the OFT and AV canal in the morphant (green and red arrowheads ing, respectively). (d–j) Other target genes,pdcd4a(d,h),pdcd4b(e,i) andptenb(f,j) were induced in the morphant (h–j). Expression of these genes was not observed in the WT (c–f). Scale bars, 50 μm (c–j). Figure 5: Sequence alignment and expression patterns of selected genes. ( a ) Sequence alignment of zebrafish miR-21 , 3′-UTR of spry2 and its mutated version is shown, with the seed sequences highlighted in yellow and the complementary nucleotides in red and green. ( b ) The EGFP-spry2 reporter with the WT spry2 3′-UTR gave strong fluorescent signals when the endogenous miR-21 was blocked by the MO against it (left panel), but failed to show the signals when co-injected with the miR-21 duplex (middle panel). The EGFP-spry2 reporter mRNA, in which the seed sequence was mutated, produced strong signals even when co-injected with the miR-21 duplex (right panel) at 24 hpf. ( c,g ) Expression of the endogenous spry2 was not observed in the WT at 72 hpf ( c ), whereas it was induced in both the OFT and AV canal in the morphant (green and red arrowheads in g , respectively). ( d – j ) Other target genes, pdcd4a ( d , h ), pdcd4b ( e , i ) and ptenb ( f , j ) were induced in the morphant ( h – j ). Expression of these genes was not observed in the WT ( c – f ). Scale bars, 50 μm ( c – j ). Full size image These results are consistent with observations that although spry2 is not normally expressed in the OFT and AV canal, it was induced in the miR-21 morphants ( Fig. 5c ), indicating that the regulatory action of miR-21 is mediated at least by inhibition of s pry2 and removal of suppression of the MAP kinase cascade. We also confirmed that expression of programmed cell death 4a ( pdcd4a ), 4b ( pdcd4b ) and phosphatase and tensin homologue B ( ptenb ) were induced in the miR-21 morphants ( Fig. 5d–f and h–j ), consistent with mouse miR-21 (refs 38 , 39 ). Hence, in both species, miR-21 acts as a positive regulator of cell proliferation. Sequence alignments of the target regions are shown in Supplementary Fig. S7 . These results were further confirmed by qRT–PCR, using RNA isolated from whole bodies expressing miR-21 as a transgene (see Supplementary Fig. S7 ). To confirm the roles of spry2 and the MAP kinase cascade, we injected a target protector MO against spry2 ( spry2 target protection (TP) MO). Protection of spry2 was confirmed (see Supplementary Fig. S8 ). At 48 hpf, the spry2 TP MO-injected embryos showed signs of pericardiac oedema and incomplete looping of the heart tube ( Fig. 6b ). Next, we treated developing embryos with U0126, an inhibitor of the MAP kinase pathway to mimic the inhibitory effect of spry2 (ref. 40 ). U0126-treated embryos showed a cardiac phenotype similar to that of the spry2 TP MO-injected embryos ( Fig. 6d ) and miR-21 morphants ( N =92/145 for the spry2 TP morphants and 56/92 for the U0126 treatment) ( Fig. 4 ). 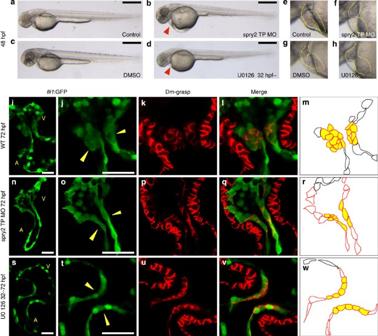Figure 6: Effects of a gain of function of spry2 and U0126 treatment. (a–h) When the MAP kinase cascade was blocked by injection of a target protection (TP) MO ofspry2(b,f) or U0126-treatment (d,h), hearts (dotted outlines) exhibited incomplete looping (f,h). Red arrowhead indicates pooling of blood, a sign of stagnation of circulation. The normal looped heart is shown in (e). (i–w) As observed in themiR-21morphants and the arrested hearts, the endocardial cells were single-layered, flattened and stretched in the hearts injected with the TP MO ofspry2(n–r) and the U0126-treated embryos (s–w). Normal thickening of cells observed in the WT (i–m) was lost, as visualized byfli1-GFPreporter and Dm-grasp staining. As illustrated in a schematic representation (m,randw), the multi-layered cuboidal cells observed in the WT (m) was detected neither in the hearts injected with the target protection MO ofspry2(r) or treated by U0126 (w). Scale bars, 500 μm (a–d), 50 μm (i,j,n,o,s,t). Figure 6: Effects of a gain of function of spry2 and U0126 treatment. ( a – h ) When the MAP kinase cascade was blocked by injection of a target protection (TP) MO of spry2 ( b , f ) or U0126-treatment ( d , h ), hearts (dotted outlines) exhibited incomplete looping ( f , h ). Red arrowhead indicates pooling of blood, a sign of stagnation of circulation. The normal looped heart is shown in ( e ). ( i–w ) As observed in the miR-21 morphants and the arrested hearts, the endocardial cells were single-layered, flattened and stretched in the hearts injected with the TP MO of spry2 ( n – r ) and the U0126-treated embryos ( s – w ). Normal thickening of cells observed in the WT ( i – m ) was lost, as visualized by fli1-GFP reporter and Dm-grasp staining. As illustrated in a schematic representation ( m , r and w ), the multi-layered cuboidal cells observed in the WT ( m ) was detected neither in the hearts injected with the target protection MO of spry2 ( r ) or treated by U0126 ( w ). Scale bars, 500 μm ( a – d ), 50 μm ( i,j,n,o,s,t ). Full size image Morphological alterations were confirmed by the green fluorescent protein (GFP) signals and Dm-grasp staining in fli1:GFP transgenic fishes at 72 hpf ( Fig. 6i–w ). In both the spry2 , TP MO-injected and U0126-treated embryos, the endocardial cells showed neither clustering nor thickening, with only a single layer of thin GFP-positive cells ( Fig. 6n–w ). As revealed by Dm-grasp staining, only a few thin cells were visible at the AV canal ( Fig. 6p–r and u–w ), whereas clustering of the multi-layered cuboidal cells was formed in the WT ( Fig. 6k–m ). We also found that the endocardial cell number at the AV canal was decreased approximately by half in both the spry2 TP MO-injected and U0126-treated embryos (see Supplementary Fig. S8 ). In both the spry2 , TP MO-injected and U0126-treated embryos, the myocardial expression of versican was expanded, whereas bmp4 was unchanged. The endocardial expression of notch1b and has2 became stronger. Expression of spp1 was suppressed (see Supplementary Fig. S9 ). PCNA staining was also suppressed (see Supplementary Fig. S5 ). Next, we examined MAP kinase signalling by staining a phosphorylated form of Erk1/2 at 55 hpf ( Fig. 7 ). In the WT, staining was evident in the cuboidal endocardial cells at the AV boundary ( Fig. 7a–c ). In the miR-21 morphants, staining was lost ( Fig. 7d–f ). When heartbeat was arrested from 24 to 55 hpf by BDM, faint signals were detected only on the luminal surface ( Fig. 7g–i ). Likewise, staining was significantly repressed in the spry2 TP MO-injected and U0126-treated embryos ( Fig. 7j–o ). These data indicate that the heartbeat, miR-21 , spry2 and MAP kinases are in the same signalling cascade. 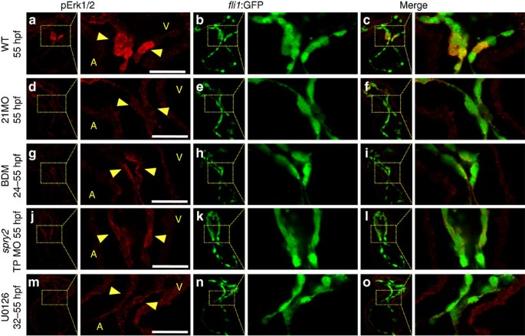Figure 7: Suppression of MAP kinase signalling inmiR-21morphants and BDM-treated hearts. (a–c) In the WT beating hearts, a phosphorylated form of Erk1/2 (pErk1/2) was stained in the cuboidal endocardial cells at the AV junction (yellow arrowheads ina). The entire endocardial cells were labelled by GFP, which expression was driven by thefli1promoter (b,c). (d–f) In themiR-21morphants, the pErk1/2 staining was week and the cells were flat. (g–i) When the heartbeat was stopped by BDM, phosphorylation of Erk1/2 was also suppressed, leaving only faint staining in the apical surface of flattened endocardial cells. (j–o) Injection of themiR-21target protection MO and the U0126 treatment gave the same results on pErk1/s staining. A, atrium; V, ventricle. Scale bars, 20 μm. Figure 7: Suppression of MAP kinase signalling in miR-21 morphants and BDM-treated hearts. ( a – c ) In the WT beating hearts, a phosphorylated form of Erk1/2 (pErk1/2) was stained in the cuboidal endocardial cells at the AV junction (yellow arrowheads in a ). The entire endocardial cells were labelled by GFP, which expression was driven by the fli1 promoter ( b , c ). ( d – f ) In the miR-21 morphants, the pErk1/2 staining was week and the cells were flat. ( g – i ) When the heartbeat was stopped by BDM, phosphorylation of Erk1/2 was also suppressed, leaving only faint staining in the apical surface of flattened endocardial cells. ( j – o ) Injection of the miR-21 target protection MO and the U0126 treatment gave the same results on pErk1/s staining. A, atrium; V, ventricle. Scale bars, 20 μm. Full size image Once contraction of cardiomyocytes commences, it continues for the entire lifetime. However, patterns of blood flow change along with transformation of the heart structures. Oxygen and nutritional demands change during development and with physiological and pathological conditions in adults so that cardiac tissues must change their structure and function accordingly. In both cardiogenesis and homoeostatic adaptation, cardiac tissues sense physical forces generated by the heartbeat and blood flow and respond with changes in gene expression. Thus, cardiac cells are mechanotransducers that convert physical inputs into biological outputs [41] , [42] . The molecular mechanisms of this signal conversion are largely unknown. Functional links between physical forces and gene expression are implied by the demonstration that the lineage of mesenchymal stem cells can be directed by matrix elasticity [43] . In the vascular system, shear stress induces Klf2 . Knock-out of mouse Klf2 results in a loss of the vascular integrity and subsequent haemorrhage, reinforcing the role of shear stress-dependent Klf2 expression in the vascular homoeostasis [44] . In zebrafish, expression of klf2a in the AV canal is dependent on reversing blood flow. A loss of function of klf2a , which can be mimicked by arresting heartbeat or injecting an MO against klf2a , results in dysgenesis of the valve [7] . These lines of evidence emphasize that physical stimuli regulate gene expression, but to date, the precise mechanisms remain to be elucidated. This report has shown that expression of zebrafish miR-21 is dependent on the heartbeat. Arrest of the heart for 12 h eliminated the expression of both the primary and mature forms of miR-21 ( Fig. 2 ). More importantly, its expression was restored by a period of heartbeat as short as 1 h ( Fig. 2 ). A similar rapid response was seen in the epinephrine-stimulated head vasculatures ( Fig. 3 ) and HUVECs stimulated by shear stress (see Supplementary Fig. S2 ). However, the induction profiles of the pri-miR-21 , mature miR-21 , KLF2 are different in HUVECs, depending on the natures of the applied flows. Endothelial cells are known to respond differently to chaotic and steady flows [45] , [46] , and the expression of zebrafish klf2a is dependent on the reversing flow, reinforcing the importance of the flow during cardiogenesis and physiological adaptation. In addition, a set of genes can be induced by the flow in a temporally controlled manner, with miR-21 , klf2a and egr1 as early responders and miR-143 and miR-23 as late ones. In this sense, it is particularly important that miR-23b and miR-143/145 can be induced by KLF2 in HUVECs [47] , and that EGR1 binds to regulatory regions of the miR-23a/24/27a cluster and KLF2 (ref. 48 ). This indicates that this hierarchical induction contributes to the distinct temporal profiles of gene induction. Recently, stress-dependent remodelling of cardiac tissues has been shown to occur in the absence of miR-21 in mouse (T.B. et al., unpublished observation) [17] , [36] , [49] . Genetic deletion of miR-21 protects against tumour formation via modulation of the MAP kinase cascade [15] but the valveless phenotype was not found in either miR-21 -null or antagomir-treated mice [15] , [17] . This implies that miR-21 acts differently in different tissue contexts (cardiomyocytes/cardiac fibroblast in mouse versus valve-forming endocardial cells in zebrafish), yet regulating the same targets. Phenotypic differences are also seen in Klf2 / klf2a . Klf2 -null mice show abnormal vascular morphology, a loss of vessel wall stability and heart failure [44] , whereas the klf2a -morphants display dysmorphogenesis of the valve [7] . The phenotypic discrepancies observed in miR-21 and Klf2 / klf2a might relate to the fact that valve leaflets arise from the mesenchyme cushion in mice, whereas they are formed by protrusion of the endocardium in zebrafish [50] . As cardiomyocytes and mesenchymal cells do not contact the blood stream, they are unable to receive flow stimuli. This spatial separation prevents them from responding to shear stress. Shear stress and stretch activate miR-21 with different temporal profiles (our unpublished observation), hereby these two stimuli could act differently. In addition, signalling cascades specifically acting on cardiomyocytes, such as BMP, might modify the actions of miR-21 , as suggested by SMAD-dependent maturation of miR-21 (ref. 51 ). We also do not exclude the possibility that myocardial contraction might affect expression of miR-21 by an unknown mechanism. In addition to these developmental contexts, the haemodynamic forces may differ between the zebrafish and mouse; for example, the Reynolds number at the valve-forming stage is 0.017 at 26 hpf in zebrafish and 0.205 at 10.5 dpc in the mouse [52] , implying that viscous shear forces are relatively more important for zebrafish cells. miR-21 is also expressed in the OFT and AV valves of adult hearts ( Fig. 1 ). In adult mammals, valves and vascular endothelial cells are susceptible to mechanical injury and pathogenic conditions associated with irregular shear, leading to cell proliferation and expression of genes, including Egr1 (refs 53 , 54 , 55 ). Accordingly, the expression miR-21 in the adult valves of zebrafish might be involved in their homoeostatic maintenance. Recently, it was shown that excessive endocardial cushions were formed in zebrafish dicer mutant [30] , a conflict result with the miR-21 morphants. However, in the dicer mutant, processing of all miRNAs are blocked not only in the endocardium, but also in the myocardium, implying that unknown miRNA(s) might be negatively involved in the formation of endocardial cushions. We have demonstrated that miR-21 is a novel component of a mechanotransduction pathway in which blood flow is the primary stimulus for gene expression. This is summarized in Supplementary Fig. S10 . In effect, physical forces act as a ‘morphogen’ producing a gradient of mechanical strain in tissues. Anisotropic distribution of strains is translated into asymmetric gene expression. Future research will look for factors shuttling between the cytoplasm and nucleus in response to mechanical stresses, that is, potential regulatory factors of miR-21 . By integrating these lines of investigation, we aim to achieve a better understanding of the physical aspects of cardiogenesis and circulatory homoeostasis and, ultimately, to develop new therapeutic methods for diseases caused by haemodynamic changes. Antibodies and reagents To change the haemodynamics, zebrafish embryos were placed in water containing 10 mM of BDM (2,3-butanedione monoxime: Sigma, B-0753) or 2 mM of epinephrine (Wako) at proper stages. For exposure to U0126 (Merck Ltd), embryos were incubated with 100 μM U0126 in 2% dimethyl sulfoxide from 32 hpf until fixation. In all experiments, embryos treated with the vehicles alone were used as a control. An antibody against pERK1/2 (1:100) was purchased from Cell Signaling Technology. Antibodies against dm-grasp (1:200), GFP (1:500) and zebrafish PCNA (1:100) were from Developmental Studies Hybridoma Bank (DSHB), Sigma and AnaSpec, respectively. cDNA probes and in situ hybridization Zebrafish in situ hybridization probes were isolated from complementary DNA (cDNA) templates using standard PCR techniques with appropriate sets of primers. To detect expression of mature miR-21 , DIG-labelled LNA probes were purchased from Integrated DNA technologies. Both whole mount and section in situ hybridization experiments were performed according to the protocol published by Exiqon [56] , [57] . Quantitative real-time PCR Approximately 20 zebrafish whole embryos, 10–15 zebrafish hearts and cultured cells (approximately 1 × 10 5 HUVECs) were homogenized with MULTI-BEADS SHOCKER (MB901U, Yasui Kikai, Osaka, Japan). Total RNAs were isolated by RNeasy Kit (Qiagen), according to the manufacturer’s instructions. Each sample was reverse-transcribed into cDNA by miScript RT Kit (Qiagen) and was subjected to qRT–PCR analysis with miScript SYBR Green PCR Kit (Qiagen). Each experiment was carried out with at least one additional biological and experimental replicate. Results in Fig. 3 and Supplementary Fig. S1–S3 are shown as mean fold changes ±s.e.m. qRT–PCR primers shown in Table 1 . Table 1 qRT–PCR primers. Full size table Immunohistochemistry and cell counting Zebrafish embryonic hearts were isolated in L-15 medium (Gibco) and fixed in 4% paraformaldehyde for overnight at 4 °C (for PCNA detection, 1 h at room temperature). Fixation solution was replaced with PBDT (1% bovine serum albumin (BSA); 0.1% Triton X-100; 1% dimethyl sulfoxide in phosphate buffered saline (PBS)) for 1 h. Fixed hearts were incubated with a primary antibody for overnight at 4 °C, briefly washed with PBDT and subsequently incubated with a second antibody conjugated with Alexa Fluor 488 or 594 and 4',6-diamidino-2-phenylindole (Sigma). Hearts were imaged using a confocal microscope (Olympus FV1000). In order to count the cell number, cell counter plugin with ImageJ was employed. For myocardial cells counting, the hspGFF3A transgenic line, which expresses myocardium-specific GFP signal, was used. fli1 :GFP transgenic line was used for counting the endocardial cells, as well as the PCNA and/or dm-grasp-positive cells. Error bars express mean ±s.e.m. and statistical significance was determined by a t -test ( P <0.05). The transgenic zebrafish lines fli1-EGFP were kindly provided by Kawahara and colleagues [58] . hspGFF3A was described previously [59] . Injection of morpholino oligonucleotides and mRNAs into zebrafish eggs MOs were designed and synthesized by Gene Tools (Philomath, OR). Initially, we made several MOs against miR-21 . One MO (5′-GCCAACACCAGTCTGATAAGCTA-3′), which was also used by Bakkers and colleagues [30] , was found to be ineffective, as injection of this MO did not induce any specific abnormality in the heart. Other MOs gave the consistent results. MOs were dissolved in the Danieau solution. Approximately 1 nl of MOs were injected into the yolk at the one-cell stage. Sequences, injection concentration and dose are as follows: miR-21-1 , Multiblocking 5′-TGTAACAGCCAACACCAGTCTGATAAGCTAT-3′ (1 mM, 10 ng) miR-21-2 , Multiblocking 5′-ACTCAAAGCCAACACCAGTCTGATAAGCTAC-3′ (1 mM, 10 ng) miR-21-1, Guide Dicer, 5′-ACAGCCAACACCAGTCTGATAAGCT-3′ (2 mM, 16 ng) miR-21-2, Guide Dicer, 5′-AAAGCCAACACCAGTCTGATAAGCT-3′ (2 mM, 16 ng) spry2 miR-21 target protector, 5′-ACTTCAAACCAGTTTTTGCCAATCC-3′ (2 mM, 16 ng) scrambled MO, Oligo-25N (2 mM, 16 ng). Sequences of klf2a , 5′-AGCTGAGATGCATGGACCTGTCCAG-3′ (2 mM, 16 ng), tnnt2 , 5′-CATGTTTGCTCTGATCTGACACGCA-3′ (0.5 mM, 4 ng), gata1 , 5′-CTGCAAGTGTAGTATTGAAGATGTC-3′ (1 mM, 8 ng), gata2 , 5′-CATCTACTCACCAGTCTGCGCTTTG-3′ (1 mM, 8 ng), and tbx2b , 5′-GAGCGTGGAAAGGGTGGTAAGCCAT-3′ (0.25 mM, 2 ng) were previously described [7] , [19] , [22] , [24] , respectively. To ensure the efficient knockdown, miR-21-1 and miR-21-2 MOs were co-injected after mixing equal amounts of two MOs. The miR-21 morphants shown in this article are by the miR-21 multiblocking MO, except for Fig. 4d . For overexpression of miR-21 , miRNA duplexes were purchased from Integrated DNA Technologies, Inc., and were resuspended in the Danieau buffer to a concentration of 100 μM. The sequences are as follows: miR-21 duplex A: 5′- UAGCUUAUCAGACUGGUGUUGGC-3′ miR-21 duplex B: 5′- GCCAACACCAGUCUGAUAAGCUA-3′. In vitro transcription of EGFP-z-spry2 3′-UTR and mCherry mRNAs were performed with mMESSGAE mMACHINE kit (Applied Biosystems) and these synthesized mRNAs were purified with G-50 Micro Columns (GE Healthcare). Generation of transgenic zebrafish lines For construction of the miR-21 expression vector, pre-miR-21 sequence was amplified by PCR from cDNA template and cloned into pT2KXIGΔin vector [60] . The Tol2 transposon-mediated transgenesis was carried out by following the procedure described elsewhere [60] . Luciferase assay HEK293T cells are transfected with psi-CHECK2 vector (Promega) harbouring z-miR-21 -binding site and the z-miR-21/GFP expression vector (pT2KXIGΔin-miR-21/GFP). miRNA dual luciferase assay was carried out by using the Dual luciferase assay kit (Promega). Shear stress experiment HUVECs were cultured with Medium 199 (Invitrogen) containing 20% fetal bovine serum (FBS) (SAFC Biosciences), 10 ng ml −1 basic fibroblast growth factor (bFGF) (Austral Biologicals) and 1% penicillin–streptomycin (Invitrogen). For experiments, HUVECs were cultured in a 35-mm plastic dish (Iwaki) pre-coated with 0.1% bovine gelatin (Sigma-Aldrich). The experiments were conducted after the cells reach confluence. For the experiments, medium was replaced with Medium 199 containing 0.5% FBS and 1% penicillin–streptomycin, and HUVECs were incubated for 2 h under static condition. For exposing HUVECs to laminar shear stress, a parallel plate flow-chamber, roller pump (HV-07523-80, Master Flex), two reservoir bottles and silicone tubes were used. One reservoir was open to the atmosphere, and the medium in the flow circuit was equilibrated with 95% air and 5% CO 2 to maintain pH. For the reciprocating flow experiments, the flow-exposure system consisting of the flow-chamber, a 50-ml syringe (Terumo) mounted on a syringe pump (KDS270, KD Scientific), a reservoir glass tube, and silicone tubes were. The flow-chamber was composed of a cell culture dish, a polycarbonate I/O unit, and a silicone gasket. The systems were maintained at 37 C. The flow channel with a length of 22 mm, a width of 14 mm and a height of 0.4 mm was used for generating shear stress of 2.0 Pa. HUVECs were exposed to laminar flow with a shear stress of 2.0 Pa or reciprocating flow with a shear stress of ±2.0 Pa and a frequency of 0.5 Hz for 15, 30, 45, 60, 120 and 240 min in the flow-chamber. Shear stress estimation The fli1a:GFP / gata1:RFP transgenic zebrafish line was mounted in low-melting agarose and treated with 2 mM epinephrine, and movies of blood circulation were taken before and 45 min after epinephrine stimulation with a high speed video camera (EX-F1, CASIO) (30 fps). Velocity of blood flow ( v ) and vessel diameters were measured by the ImageJ software (15 embryos on average). Velocity of blood flow was estimated from migration speed of three RFP-marked blood cells’ centroid in two frames. Average vessel diameter ( a ) was obtained from three different points of GFP marked-vessel endothelial cells. The shear stress ( τ ) is τ=4μQ/πa [3] . Q is the volumetric flow rate and we postulated that Q is equal to v in this estimation. We assumed that blood viscosity ( μ ) is not altered in the presence of epinephrine. Hence, shear stress ratio of epinephrine treated embryos ( τ 45 ) to untreated ( τ 0 ) can be given by τ 45 /τ 0 . Error bars represent mean ±s.e.m. Statistical significance was determined by a t -test ( P <0.05). How to cite this article: Banjo, T. et al. Haemodynamically dependent valvulogenesis of zebrafish heart is mediated by flow-dependent expression of miR-21 . Nat. Commun. 4:1978 doi: 10.1038/ncomms2978 (2013).